A quantitative analysis of transmission efficiency versus intensity for malaria The relationship between malaria transmission intensity and efficiency is important for malaria epidemiology, for the design of randomized control trials that measure transmission or incidence as end points, and for measuring and modelling malaria transmission and control. Five kinds of studies published over the past century were assembled and reanalysed to quantify malaria transmission efficiency and describe its relation to transmission intensity, to understand the causes of inefficient transmission and to identify functions suitable for modelling mosquito-borne disease transmission. In this study, we show that these studies trace a strongly nonlinear relationship between malaria transmission intensity and efficiency that is parsimoniously described by a model of heterogeneous biting. When many infectious bites are concentrated on a few people, infections and parasite population structure will be highly aggregated affecting the immunoepidemiology of malaria, the evolutionary ecology of parasite life history traits and the measurement and stratification of transmission for control using entomological and epidemiological data. Malaria, dengue, filariasis and other mosquito-borne diseases cause several hundred million cases of clinical disease and more than one million deaths each year. A theory of mosquito-borne disease transmission and control has been developed around a mathematical model described by Ross, analysed by Lotka, and parameterized and applied by Macdonald [1] , [2] , [3] . The theory describes the potential intensity of transmission and the dynamics of mosquito-borne diseases in terms of the basic reproductive number R 0 , the number of infectious mosquitoes that would arise from a single infectious mosquito after one parasite generation in an immunologically naive population [2] , [4] . A formula for R 0 is based largely on entomological aspects of transmission described by vectorial capacity, the number of infectious bites that would eventually arise from all the mosquitoes that bite a fully infectious human on 1 day [5] . R 0 describes a threshold for endemic persistence of malaria and other weakly immunizing mosquito-borne infections, a threshold for epidemic spread of strongly immunizing pathogens, the rate of increase in the number of cases during an epidemic [6] and a basis for setting transmission reduction targets that must be achieved through vector control to eliminate endemic transmission or prevent epidemics [4] , [7] , [8] . R 0 can be estimated directly through entomological studies and vectorial capacity, or it can be estimated indirectly using epidemiological, serological or entomological measures of transmission [4] , [9] . Two serious challenges to the quantitative validity of using entomological metrics for control were raised by studies that obtained very different indirect estimates of R 0 using different measures of transmission [10] , [11] . One measure of transmission is the average number of infectious bites per person per unit time, called the entomological inoculation rate (EIR). Another measure of transmission is the number of infections per person per unit time, called the force of infection (FOI). The FOI counts all incident (that is, new) human malaria infections in some time interval with or without clinical symptoms, and whether or not a person is already infected. The number of infections per infectious bite (FOI/EIR) describes the efficiency of transmission. A third measure of transmission is the sero-conversion rate (SCR), the rate that humans develop serological responses to the products of parasite infections; the SCR is analogous to the FOI and would be very similar if serological responses were highly predictive of previous infection. Several studies that have estimated transmission efficiency have shown that malaria transmission is extremely inefficient in high-intensity settings [10] , [12] , [13] , [14] , [15] , [16] , [17] , [18] , and there has been a long-standing debate about why [17] , [18] , [19] , [20] , [21] , [22] . Low transmission efficiency gave rise to the challenges about the quantitative validity of using entomological measures as a basis for measuring transmission and planning control. One reason for inefficient malaria transmission is that the parasites may not be transmitted from an infectious mosquito to a human during the blood meal. Once in a human or other vertebrate host, transmitted sporozoites could also fail to advance to the blood stages by chance. Some infections may be prevented by an acquired pre-erythrocytic immunity to malaria, but despite evidence that immunity to pre-erythrocytic stages can be induced artificially, there is very little direct evidence that pre-erythrocytic immunity blocks a high fraction of incoming infections [23] . Immunity to blood stages of the parasites, especially in those who have well-developed blood-stage immunity, could also cause inefficient transmission by rapidly clearing primary merozoites or suppressing parasite densities below levels that are detectable by microscopy, thereby preventing patent (that is, detectable) infections [19] , [24] . It has also been proposed that an acute immune response to mosquito bites could confer short-term protection against infection [25] . A variety of other explanations have been proposed to explain inefficient transmission in infants, such as fetal haemoglobin, changes in the intestinal flora, the predominance of a milk-based diet and maternal antibodies, but these would not explain inefficient transmission observed in older children [20] . Another explanation is heterogeneous biting, in which a few people receive most of the infectious bites [18] , [26] , [27] . Contrast homogenous biting, in which 10 different people each get 1 infectious bite, with heterogeneous biting, in which 1 infectious person gets 10 infectious bites and the other 9 get none. Infections are not directly observable, so by most methods, heterogeneous biting would make it appear that there are many fewer infections than infectious bites. Transmission would also appear to be inefficient if the estimates of the EIR were biased, such that estimates of the EIR were always higher than the actual EIR. The critical issues are the degree of transmission efficiency, its quantitative relationship to the EIR, and the underlying cause of the apparent transmission inefficiency, whether it is heterogeneous biting, immunity or measurement bias. These causes are not mutually exclusive; each factor could explain some part of the discrepancy. What remains unclear is what the apparent inefficiency of malaria transmission means for the control of malaria and other mosquito-borne diseases. Two key assumptions of the basic theory of mosquito-borne transmission are that the potential intensity of transmission is related to the vectorial capacity [5] , and that the number of human infections that occurs is proportional to the number of infectious bites. The studies of malaria provide a chance to test the mosquito-based theory to evaluate whether the cause of inefficient transmission is likely to be unique to malaria, or whether these same patterns would likely apply in other settings and to other mosquito-borne diseases. In this study, we have assembled and analysed malaria data to look for broad patterns, such as systematic differences in the efficiency of transmission across the spectrum of transmission intensity. The assembled data trace a strongly nonlinear relationship between transmission efficiency and transmission intensity; the number of infectious bites ranged up to several hundred per year, but the number of infections rapidly saturates when the annual EIR is >10. The patterns suggest that immunity does not explain inefficient transmission in young children, but that a model of heterogeneous biting does. These results will affect the way commonly measured malaria metrics are used to stratify transmission to plan for and evaluate the outcome of malaria control programmes. Literature search A preliminary literature search identified five kinds of studies that estimated transmission efficiency either directly by exposing people to the bites of infectious mosquitoes, or indirectly as the ratio of the FOI and the EIR, the number of infections per infectious bite: (1) human subjects were challenged by exposing them to the bites of infectious mosquitoes [28] , [29] , [30] , [31] ; (2) synthetic cohorts of uninfected people were created by curing infections with antimalarial drugs, and the cohorts were followed over time to estimate the attack rate: the proportion of the cohort that was infected [16] , [32] , [33] ; (3) cross-sectional parasite surveys were used to estimate the FOI by fitting models to the rise in malaria prevalence with age, after accounting for infections that were cleared [12] , [13] , [14] ; (4) cross-sectional serological surveys were used to estimate the SCR by fitting models to the rise in seroprevalence with age, after accounting for waning immunity (or sero-reconversion) [34] , [35] ; and (5) longitudinal studies were used to estimate the FOI by following individuals over time as they naturally acquired infections, and several study designs and methods were used to infer the attack rates from a sequence of parasite positive or negative observations [15] , [36] , [37] . These studies were reanalysed and the results assembled to evaluate the functional relationship between the FOI (denoted h in equations, which Ross called the 'happenings' rate [1] ) and the EIR (denoted E in equations). The efficiency of transmission (that is, h/E ) was also plotted as a function of the EIR. Experimental challenge One source of the discrepancy between the EIR and the FOI is the proportion of infectious bites that cause a patent infection in a population previously unexposed to malaria, denoted as b . A nearly ideal natural experiment to estimate b has been conducted ethically by experimental challenge to infectious mosquitoes in the non-intervention arms of drug or vaccine trials on subjects who had no previous malaria exposure [29] , [30] , [31] . 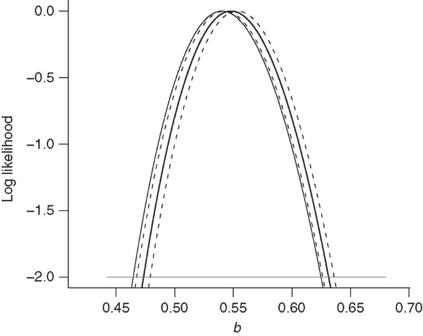Figure 1: The log likelihood of the proportion infected per bite after experimental challenge to infectious mosquitoes. Data were assembled from the non-intervention arms of vaccine and drug trials in carefully monitored studies using human subjects previously unexposed to malaria (Table 1). The thin solid line uses only the data for which an exact number of infectious bites were reported. The two dashed lines use the upper or lower bound or the upper bound for the number of infectious bites. The solid line uses the average of the log likelihood from the upper and lower bound. In people previously unexposed to malaria, the ratio of the FOI to the EIR is∼55%, with confidence limits between 47 and 63%. Data from these trials were assembled and analysed ( Table 1; Supplementary Note 1 ). Table 1 The outcome of experimental challenge to the bites of infectious mosquitoes. Full size table The analysis assumed independent infection probabilities: the probability of infection after being challenged with n infectious bites was 1−(1 −b ) n . Some trials report a range for the number of infectious mosquitoes in the challenge, so maximum likelihood analysis to estimate b was performed in four ways ( Fig. 1 ). Maximum likelihood estimation (MLE) estimates of b were as follows: 54% (47–62%) using only those data that reported the exact number of challenge mosquitoes; 55% (64–48%) using the lower bound on the number of bites; 54% (47–63%) using the upper bound on the number of bites; and 55% (47–63%) by averaging the log likelihood of the lower and upper bounds. Figure 1: The log likelihood of the proportion infected per bite after experimental challenge to infectious mosquitoes. Data were assembled from the non-intervention arms of vaccine and drug trials in carefully monitored studies using human subjects previously unexposed to malaria ( Table 1 ). The thin solid line uses only the data for which an exact number of infectious bites were reported. The two dashed lines use the upper or lower bound or the upper bound for the number of infectious bites. The solid line uses the average of the log likelihood from the upper and lower bound. In people previously unexposed to malaria, the ratio of the FOI to the EIR is ∼ 55%, with confidence limits between 47 and 63%. Full size image A synthetic cohort study Analysis of synthetic cohorts was carried out in Saradidi, Kenya, in 1986–1987 to provide baseline epidemiological information prior for a vaccine control trial [16] . Every month, a new cohort of ∼ 40 children was drawn at random from the whole population, and their malaria infections were cleared with the antimalarial drug sulphadoxine–pyrimethamine. After waiting a month until the drugs had cleared, the cohort was followed for 2 more months. The EIR was measured by human landing catches in each 2-week period and it was then compared with the attack rate: the proportion of the population that became infected in the subsequent 2-week period. Variability in the EIR over 44 consecutive 2-week periods was reflected in variable incidence in the 21 different cohorts, and this provided a way of estimating transmission efficiency over time, while the daily EIR was measured at values ranging from zero up to five infectious bites per person per day. Three models were fit to these data. First, the FOI in a population with a given EIR and a fixed level of immunity would be given by the equation h = bE ; this is the assumption made by the Ross–Macdonald model. Second, in the original study from Saradidi, the data were described by a linear relationship: h = h 0 + bE . This unrooted linear model thus predicts that transmission still occurs at the rate h 0 even when the EIR is actually zero. Third, heterogeneous biting could explain the observed relationship between the EIR and the FOI [18] . With Gamma -distributed biting rates (Methods), a nonlinear relationship between the EIR and the FOI is given by the equation: When biting is more heterogeneous, the estimated FOI is lower relative to the EIR. 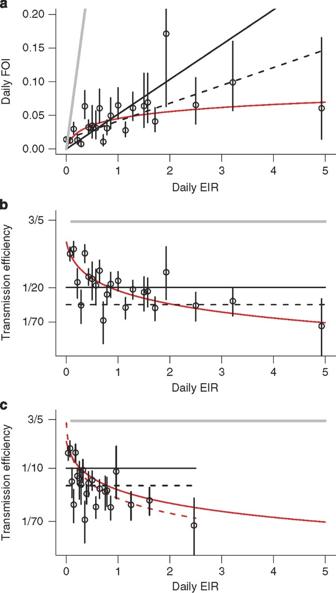Figure 2: Data and fitted models from the reanalysis of the synthetic cohort study. The top two panels have replotted the original data and results of the reanalysis in two ways: (a) the daily FOI and (b) transmission efficiency versus the daily EIR. Each point is an estimate of the daily FOI or transmission efficiency; the bars show the confidence intervals on the FOI by the exact test on the attack rate. Lines show the best fits for the fitted models: solid black is the rooted linear model (b≈1/20), dashed black shows the slope from the unrooted linear model (b≈1/37) and red shows the best-fit heterogeneous biting model. The grey line is plotted for reference to show the relationship predicted by the Ross–Macdonald model (that is, a linear relationship), assumingb=0.55. (c) Under the assumption that EIR was biased by a factor of two, the analysis was redone and plotted as transmission efficiency. The fitted slopes for the rooted (solid black) and unrooted (dashed black) linear models are different (b≈1/10 or 1/20, respectively). The dashed red line shows the new best fit for the heterogeneous biting model. The solid red line and grey lines were replotted frombfor reference. The linear models and Equation 1 were fitted to the data from Saradidi using MLE and ranked by Akaike's information criterion (AIC, Table 2 , Fig. 2 ). The rooted linear relationship fits very poorly. The unrooted linear function provides the best fit to the data; the fitted values could be interpreted to mean that the actual EIR was less variable and more like the overall average in the synthetic cohort compared with the estimated EIR. Table 2 Results of the reanalysis of the synthetic cohort study. Full size table Figure 2: Data and fitted models from the reanalysis of the synthetic cohort study. The top two panels have replotted the original data and results of the reanalysis in two ways: ( a ) the daily FOI and ( b ) transmission efficiency versus the daily EIR. Each point is an estimate of the daily FOI or transmission efficiency; the bars show the confidence intervals on the FOI by the exact test on the attack rate. Lines show the best fits for the fitted models: solid black is the rooted linear model ( b ≈1/20), dashed black shows the slope from the unrooted linear model ( b ≈1/37) and red shows the best-fit heterogeneous biting model. The grey line is plotted for reference to show the relationship predicted by the Ross–Macdonald model (that is, a linear relationship), assuming b =0.55. ( c ) Under the assumption that EIR was biased by a factor of two, the analysis was redone and plotted as transmission efficiency. The fitted slopes for the rooted (solid black) and unrooted (dashed black) linear models are different ( b ≈1/10 or 1/20, respectively). The dashed red line shows the new best fit for the heterogeneous biting model. The solid red line and grey lines were replotted from b for reference. Full size image The heterogeneous biting model ranked second, but with a low ΔAIC value. The MLE of α ≈4.6 (confidence interval (CI): 3.9–5.4) corresponds roughly to the proposed rule that 20% of the population receives 80% of the bites [26] , [27] . The MLE of b was 27% (CI: 21–35%, Fig. 2b ), approximately one-half of the value found using the vaccine-trial data. In Saradidi, when only one infectious bite was counted during a 2-week period (the lowest positive count), 63/392 people (16.1%, CI: 12.6–20.1%) were infected in the subsequent 2-week period. Notably, when the EIR was estimated to be zero in the previous 2-week period, 63/349 people were infected for an attack rate of 18.1% (CI: 14.2–22.5%). A sensitivity analysis considered the potential effect of EIR measurement bias on the parameter estimates (Methods). A bias of 2 is in line with the analysis from the experimental challenges ( Fig. 2c ). Models were also developed to test the idea that short-term immunity was affecting the outcome by looking for an effect of the EIR in the previous 2–4, 4–6, 6–8 and 8–10 weeks. The model fits suggested a slightly protective effect associated with biting 6–8 weeks previously, but not with biting 2–6 weeks or 8–10 weeks previously. Cross-sectional parasite surveys Some of the most readily available data for estimating the FOI comes from cross-sectional parasite surveys that report the prevalence of infection, also called the parasite rate (PR), highly stratified by age in children <2 years [12] , [14] , [19] . A search found 23 suitable studies with paired estimates of the EIR ( Supplementary Note 2 ). The age-stratified PR data were then analysed by fitting simple 'catalytic' models using maximum likelihood (Methods). The estimates of FOI and transmission efficiency plotted with respect to the EIR revealed a similar pattern to that found in the synthetic cohort study ( Fig. 3 ). The FOI saturates when the annual EIR exceeds ∼ 10, so there is also a sharp decline in transmission efficiency. This pattern is also a robust property of the heterogeneous biting model. To demonstrate a correspondence between the shape of the heterogeneous biting model and the observed pattern, a model fitting exercise was performed with the heterogeneous biting model ( Fig. 3 , Methods). The model of heterogeneous biting describes the scatter between the EIR and the crude estimates of the FOI with the MLE parameters from the Saradidi study and t =43 days. 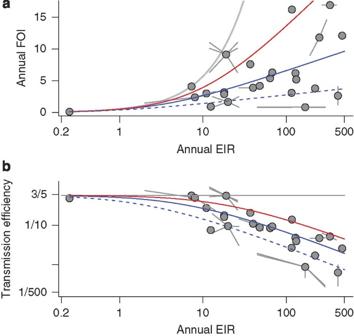Figure 3: The annual FOI and transmission efficiency estimated from cross-sectional PR surveys. The data have been plotted in two ways: (a) the estimated annual FOI and (b) transmission efficiency plotted versus the log of EIR. Each point represents a single study. When several estimates of the EIR or the FOI were reported, a 'spider' was plotted with its centre at the arithmetic mean and legs that connect the center to each one of the estimates. The solid blue line shows a good fit to the data using Equation 1, plotted withb=0.55,α=4.6 andt=43 days. The dashed blue line was drawn with longer times and much higher degrees of heterogeneous biting (that is, withα=10 andt=60 days). Also plotted in red is the heterogeneous biting model fitted to the synthetic cohort study, which serves as an upper bound for this data. The grey line is plotted for reference to show the relationship predicted by the Ross–Macdonald model, assumingb=0.55. Figure 3: The annual FOI and transmission efficiency estimated from cross-sectional PR surveys. The data have been plotted in two ways: ( a ) the estimated annual FOI and ( b ) transmission efficiency plotted versus the log of EIR. Each point represents a single study. When several estimates of the EIR or the FOI were reported, a 'spider' was plotted with its centre at the arithmetic mean and legs that connect the center to each one of the estimates. The solid blue line shows a good fit to the data using Equation 1, plotted with b =0.55, α =4.6 and t =43 days. The dashed blue line was drawn with longer times and much higher degrees of heterogeneous biting (that is, with α =10 and t =60 days). Also plotted in red is the heterogeneous biting model fitted to the synthetic cohort study, which serves as an upper bound for this data. The grey line is plotted for reference to show the relationship predicted by the Ross–Macdonald model, assuming b =0.55. Full size image Cross-sectional serological surveys Serology and parasitology were measured in cross-sectional surveys of 21 populations, and for the same populations the EIR was either measured or inferred as a function of elevation [34] . These studies thus provide a unique opportunity to examine serology and to compare it directly with parasitology. The SCR was estimated in children between the age of 1 and 10 years by looking at the proportion of individuals who were positive for at least one of the three serological markers: AMA, MSP1 or MSP2 ( Fig. 4 , Methods) [35] , [38] . 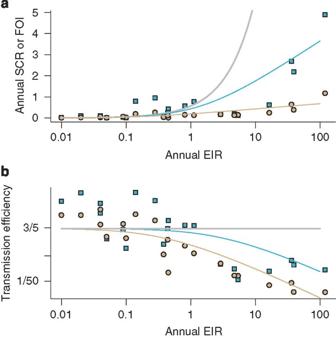Figure 4: Analysis of a set of linked cross-sectional serological and parasite surveys. The data have been plotted in two ways: (a) the estimated annual SCR (tan circles) and FOI (cyan squares) and (b) transmission efficiency based on these estimates plotted versus the log of EIR. The tan line (SCR) was plotted withb=0.55,α=4.6 andt=2 years, and the cyan line (FOI by PfPR) was plotted withb=0.55,α=4.6 andt=0.25 years. Also plotted is the predicted relationship from the Ross–Macdonald model, assumingb=0.55 (grey). Figure 4: Analysis of a set of linked cross-sectional serological and parasite surveys. The data have been plotted in two ways: ( a ) the estimated annual SCR (tan circles) and FOI (cyan squares) and ( b ) transmission efficiency based on these estimates plotted versus the log of EIR. The tan line (SCR) was plotted with b =0.55, α =4.6 and t =2 years, and the cyan line (FOI by PfPR) was plotted with b =0.55, α =4.6 and t =0.25 years. Also plotted is the predicted relationship from the Ross–Macdonald model, assuming b =0.55 (grey). Full size image In principle, the SCR is analogous to the FOI, but the two measures would only be expected to correspond if every infection generated an immunological response to the antigen(s) being tested. If immunity is heterogeneous, that is, if some individuals do not respond to the focal antigen, then the SCR will be lower than the FOI when measured by a single antigen, but for homogeneous serological responses or for a sufficiently large panel of heterogeneous serological responses, the SCR and the FOI should correspond. Notably, the estimates of SCR using a response to at least one of three markers were higher than the published estimates of the SCR using only MSP1 (ref. 34 ). In these studies, seroprevalence in children was higher than prevalence, but estimates of the FOI were, on average, five times higher than the estimates of SCR. Serology in principle provides a robust marker of previous infection, after considering heterogeneous immunity, because the decay of an immunological response is slow [34] , especially compared with infections that clear relatively quickly. With heterogeneous immunity, higher seroprevalence can produce lower estimates of SCR compared with the estimates of the FOI because parasite clearance rates ( r ≈ 1.8 per year) are ∼ 100 times higher than the estimated decay of seropositivity ( λ ≈ 0.017 per year for MSP1) [34] . The model of heterogeneous biting was fit to the data by finding a time interval, as performed above. Good fits were found with t =2 years (SCR) and 0.25 years (FOI). Other longitudinal studies In addition to the synthetic cohort studies, other longitudinal studies have estimated attack rates by following individuals over time as they naturally acquired and cleared infections. One longitudinal study in Idete, Tanzania, followed children <1 year of age for 2 weeks [36] ; attack rates were computed from individuals who were initially negative for parasites. Another longitudinal study conducted in Garki, Nigeria, followed individuals over time as they naturally acquired and cleared infections, and these data were used to estimate the FOI and the clearance rate [15] . A third study visited 94 children in Dielmo village, Senegal, every day over 4 months; all malaria attacks were observed and treated [37] . Depending on how a longitudinal study has been carried out, the estimates are prone to detection errors because parasite densities vary over the course of an infection affecting the sensitivity and specificity of microscopy [15] , [36] . Medical interventions can also interfere with the estimates if, for example, residual drug levels delay new attacks [37] . Despite the caveats, the data have been plotted without further analysis for comparison; they are broadly consistent with each other and with the other studies ( Fig. 5 ). 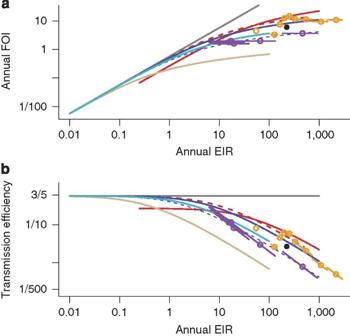Figure 5: Estimated annual FOI and transmission efficiency from all the studies plotted versus annual EIR. The data have been plotted in two ways: (a) FOI data from three longitudinal studies in Idete (orange), Garki (purple) and Dielmo (black) have been plotted without further analysis versus the annual EIR on log-log scale and (b) transmission efficiency was also plotted for those same studies. Also plotted are the Ross–Macdonald model assumingb=0.55 (grey), the reanalysis of the synthetic cohort study (red, seeFigure 2), the fit to the estimated FOI from the cross-sectional PR surveys (blue, seeFigure 3) and the fits to estimated FOI and SCR from the paired cross-sectional surveys (cyan and tan, seeFigure 4). Figure 5: Estimated annual FOI and transmission efficiency from all the studies plotted versus annual EIR. The data have been plotted in two ways: ( a ) FOI data from three longitudinal studies in Idete (orange), Garki (purple) and Dielmo (black) have been plotted without further analysis versus the annual EIR on log-log scale and ( b ) transmission efficiency was also plotted for those same studies. Also plotted are the Ross–Macdonald model assuming b =0.55 (grey), the reanalysis of the synthetic cohort study (red, see Figure 2 ), the fit to the estimated FOI from the cross-sectional PR surveys (blue, see Figure 3 ) and the fits to estimated FOI and SCR from the paired cross-sectional surveys (cyan and tan, see Figure 4 ). Full size image Cross-study comparisons The data from the longitudinal studies have been plotted along with the Ross–Macdonald model, the trend lines from the synthetic cohort study, the cross-sectional parasite surveys and the cross-sectional serological surveys ( Fig. 5 ). Across the spectrum of transmission intensity, the assembled data show that transmission efficiency varied enormously, associated strongly, negatively and nonlinearly with the EIR and differed systematically depending on the method used to measure it. Under the ideal conditions of experimental challenge in previously unexposed humans, ∼ 55% of infectious bites caused an infection (roughly half). In the synthetic cohort study, ∼ 5% of infectious bites produced an infection (that is, 1 in 20), but efficiency varied from ∼ 20% down to 1.4% (that is, from 1 in 5 to 1 in 70), and there was a nonlinear association with the EIR [16] . Highly variable estimates were found when the FOI was estimated using cross-sectional parasite surveys. An extreme estimate was ∼ 0.3% of infectious bites producing an infection (that is, 1 in 350). Very similar patterns were found in longitudinal studies. Finally, for the same EIR, transmission efficiency was lower in the serological studies by a factor of five. All these patterns arise because the annual FOI saturates at high values of the EIR, so that there were at most 15 infections per person per year. The difference between the EIR and the FOI has been measured, rediscovered and discussed several times [12] , [14] , [17] , [19] , [20] . Here, estimates of the EIR and the FOI have been assembled to show that there is a robust pattern between transmission efficiency and intensity, that the quantitative effect is large and that it is important for understanding and modelling transmission. Patterns in the assembled data raise three questions: what explains the strong association between transmission intensity and transmission efficiency; what explains the systematic differences in the estimates of transmission efficiency obtained through different methods; and finally, what explains the variability among studies? There are three dominant and non-exclusive hypotheses for the association between transmission efficiency and the EIR: immunity, heterogeneous biting and systematic bias in the estimation of the EIR. Bias in estimating the EIR could explain some of the pattern; several common methods of estimating the EIR are known to be biased relative to one another [39] , [40] . A bias in EIR could explain why the highest transmission efficiency in Saradidi was approximately half of that observed for experimental challenge to infectious mosquitoes. In that study, adults were used as bait to attract and trap the mosquitoes, but attack rates were measured in children; an observed correlation between body size and biting rates is of the right magnitude to explain the gap [41] , [42] . A similar bias would also affect the other studies. A bias in the EIR could only explain the nonlinear patterns in transmission efficiency if the magnitude of the bias increased sharply with the EIR. The studies assembled and analysed here cannot test whether such a systematic bias exists. It is possible, on the other hand, to form stronger conclusions about the relative merits of immunity. In particular, long-lasting immunity does not seem to be the main reason why transmission is inefficient. In the Saradidi study reanalysed here, in cohorts drawn at random from the same population but started at different times, transmission efficiency varied every 2 weeks and it was correlated with the EIR. Long-lasting immunity would not predict any association between transmission efficiency and the time of year when a random cohort was drawn. Other studies have come to similar conclusions about the lack of infection blocking immunity early in childhood [17] , [43] , although it might still develop in adults [17] . Blood-stage immunity is unlikely to be a factor in the young children considered in these studies, but it could be a factor in older children or adults: one study found that malaria attacks were less common in older children [37] , but another found very similar attack rates in children and adults [32] , [33] . An acute immune system response, such as to mosquito biting, could explain the variability in transmission efficiency. Curiously, estimates of the EIR 6–8 weeks previously were weakly associated with transmission efficiency, but there was no association with the EIR 2–6 or 8–10 weeks previously. In sum, immunity does not seem to explain inefficient transmission in very young children. Heterogeneous biting provides a simple, plausible and parsimonious explanation for some part of the nonlinear relationship between the EIR and the FOI. A model of heterogeneous biting, where 20% of the population gets 80% of the bites, is consistent with the EIR-correlated temporal variability in transmission efficiency observed in Saradidi, and with the patterns of transmission efficiency and intensity observed across the range of other studies described here. Heterogeneous biting also parsimoniously explains the empirical relationship between the EIR and the PR in older children [27] . Enormous variability in transmission efficiency relative to transmission intensity could be attributed to the degree of heterogeneous biting, or to a range of other factors, including the methods used to estimate the EIR or the FOI. Estimates of the EIR differ in predictable ways, depending on the methodology and frequency with which human biting rate and sporozoite rate are measured [39] , [40] , [44] , [45] , [46] , [47] . An additional explanation for the variability is that the efficiency of transmission differs among vector species [48] . The experimental challenges were almost universally conducted with infectious Anopheles stephensi , but most of the studies were conducted in Africa, where the An. gambiae complex predominates. One study, which was conducted in Madang, Papua New Guinea, had different vectors and extremely low efficiency of transmission. The Madang study was also the only study conducted, where Plasmodium vivax was highly prevalent, and, of all the studies, it had the most inefficient transmission. The lowest transmission efficiency was found using serological data, a pattern that gave rise to one of the challenges to the theory [11] . The analysis of the SCR by one of three different antigens produced higher estimates than the analysis for any one antigen, consistent with human immune responses that are highly heterogeneous: humans in a population often have a measurable serological response to some antigens but not others (that is, AMA positive, but MSP1 negative). A more relevant measure in this case may be the immune response to whole parasite antigens (either intact or lysed) rather than specific antigens. The more pressing question for this study is whether heterogeneous immunity to malaria is sufficient to explain the range of immune responses and the levels of transmission efficiency that were observed. Heterogeneous biting has broad implications for malaria epidemiology and control, for the evolutionary ecology of malaria parasites and for other mosquito-borne diseases. Aggregated exposure leads to superinfection, which could also affect other mosquito-borne diseases with multiple circulating serotypes, such as dengue. Associated parasite populations will tend to be highly aggregated among humans, and infections will be highly genetically diverse affecting parasite population genetics and parasite life history traits, including gametocytogenesis, the evolution of resistance to antimalarial drugs and the evolution of virulence. Heterogeneous biting potentially confounds every measure of malaria in epidemiology and public health, from estimates of the burden of malaria to individual risk factors for clinical or severe malaria. When exposure to malaria within a defined study population is heterogeneous, it may be possible to find individuals in that population from across the entire spectrum of exposure to malaria. If the epidemiological effects of high exposure saturate in individuals, then the functional effects of heterogeneous distributions of exposure can be larger than the effect of the average level of exposure; for example, if the risk of severe malaria and mortality were similar for children receiving either 10, 100 or 1,000 infectious bites in a year, then the incidence of severe malaria and malaria mortality in a population would be proportional to the number of children receiving more than 10 infectious bites per year. Populations with the same average levels of exposure can thus have very different outcomes, and populations with very different average levels of exposure can have very similar outcomes. Exposure to malaria has consistently been proposed as a cause of immunoepidemiological patterns and clinical outcomes of malaria across the transmission intensity spectrum [22] , [49] , [50] , for example, but similar to the relationship between the EIR and the FOI described here, the empirical relationships are highly variable and saturate at high intensity [51] . Heterogeneous biting could also be an underlying cause of the variability in measures of malaria disease and burden. The discrepancy between the EIR and the FOI is historically important and relevant for malaria transmission dynamics and control, because metrics of malaria transmission are used to stratify risk, plan for control and evaluate the responses to control. In fact, many of these studies assembled here were performed to establish baseline patterns of transmission to prepare for vaccine trials. Malaria transmission models provide a coherent framework for describing the nonlinear relationships among malaria metrics and the reductions in transmission that are required to achieve the objectives of malaria control or elimination. For control, a useful metric is the basic reproductive number, R 0 , which describes reductions in transmission required to control and ultimately eliminate malaria [4] , [8] , [9] . Practical methods for estimating R 0 rely on having malaria transmission models that can accurately describe the relationships among the most commonly measured metrics of malaria across the natural spectrum of transmission intensity, such as the PR, the EIR, the FOI or the SCR [4] , [8] , [9] . An often-overlooked aspect of transmission models is the high variability in mosquito population densities over space and time that contribute to highly focal transmission and heterogeneous biting. In this study, we have shown that the assumptions of the Ross–Macdonald model are violated, and the predictions are highly inaccurate when the EIRs exceed more than approximately one infectious bite per person per year. Because measures of the EIR are systematically much higher than the measures of the FOI, estimates of R 0 based on the EIR are much higher than the estimates based on the FOI. The enormous discrepancy between isolated estimates of R 0 made by the EIR and the FOI raised questions about the quantitative validity and utility of a vector-based theory of transmission [10] , [11] . Our analysis suggests that the discrepancy between the FOI and the EIR is to be expected and that the two metrics are consistent under a model of heterogeneous biting. The analysis also suggests that heterogeneous biting explains some part of the discrepancy between the SCR and the EIR after additionally considering heterogeneous immunity. Simple mathematical models and comparative studies can help provide a solid theoretical basis for measuring and interpreting the transmission intensity of mosquito-borne diseases using standard metrics, such as the EIR, the PR and the SCR. The standard interpretation of R 0 will need revision, however, with new modelling frameworks that consider the causes and patterns of heterogeneous biting. The data assembled in this study suggest that entomological measures and the associated estimates of R 0 still serve as a guideline for setting vector control targets, but that entomological and epidemiological measures deviate when the EIR exceeds approximately one infectious bite per person per year. R 0 may not describe the expected number of people who would be infected after one parasite generation or the rate of increase in the number of cases during an epidemic because the infectious bites are inefficiently distributed [4] . Models do, however, provide an indispensable tool for integrating information and leveraging further insight from large databases of parasite prevalence [52] when combined with methods for reconstructing the history of transmission [34] to provide an evidence-base and theoretical support for making decisions across the spectrum, from endemicity to the interruption of transmission [53] . Literature search A search was developed from a core set of papers and expanded using PubMed. The core papers were a review by Epstein et al . [29] ; the study from Saradidi, Kenya, by Beier et al . [16] ; historical papers estimating the FOI from age-prevalence relations [14] , [19] ; a recent review of studies that reported both the EIR and the PR [54] ; a published description of EIR versus SCR [34] ; and a longitudinal study conducted during the Garki project [15] . Search criteria were expanded to find other kinds of studies that had estimated malaria incidence by using a combination of terms, including 'malaria attack,' 'malaria incidence', 'entomological' and 'force of infection.' The five categories were finalized, and search methods turned to expanding the list of papers within each category. The R code used to generate all of the figures is freely available upon request. Experimental challenge Data in Table 1 were assembled starting from recent reviews [28] , [29] , [30] , [31] to find a complete set of individuals challenged to the bites of infectious mosquitoes. The search process and data sources are in the Supplementary Information . When a study reported the exact number of bites, it was considered to be both the upper and the lower bound. A synthetic cohort study Data from Beier et al . [16] were extracted to obtain the number in each cohort during each observation period, and the number that became positive. The proportion of a cohort that was positive is called the attack rate. In a homogeneous population stratum, the FOI is the hazard rate for infection, and it is related to the attack rate, A (the proportion of a cohort that becomes infected after t days) by the formula A(t)= 1 −e −ht . The FOI, h , can be computed from an attack rate by taking the inverse relationship: When biting is heterogeneous, the daily EIR varies and defines a different relationship between the FOI and attack rates. The heterogeneous biting model used here assumes that biting weights (that is, ω ) have a Gamma distribution with a mean of one and a variance of α . The biting rates, therefore, would have a Gamma distribution with the mean EIR and a squared coefficient of variation α , called the index of heterogeneous biting. After t days, the proportion of a cohort that was infected is: Observations were omitted from the analysis if the observed EIR was zero; likelihood returned an error when predicted attack rates were exactly zero but observed attack rates were positive. To account for extra-binomial variation in attack rates, the log likelihood for a set of model-based predicted probabilities, { x i }, given the corresponding sets of { P i } positive and { N i } negative observations was computed using the function: where β is the two-parameter family of beta-binomial probability distribution functions. The parameter θ is fitted along with the function that predicts { x i }, the predicted attack rates for the data from Saradidi, Kenya. The AIC (−2* LL +2 k , where k is the number of parameters) was used to compare the fits of different approximating models [55] . The MLE was repeated by assuming that the synthetic cohort experienced a real EIR that was a factor δ lower than the estimated EIR. The putative bias, δ , was varied between 1 and 10. Increasing δ initially increases the estimate of b , but after b reaches a maximum value, then a further increase in δ reduces the estimates of α , indicating less biting heterogeneity. The analysis was also repeated with the formula EIR=EIR 1 +ξ EIR 2 , where the EIR in the previous 2 weeks was called EIR 1 , and the EIR in a previous 2-week period was called EIR 2 . The heterogeneous biting model that considered the EIR 6–8 weeks before had parameter values of b =0.71, α =6.6, ξ =−0.05, θ =11.4, and it ranked higher than the model that did not consider EIR in previous periods, which had a ΔAIC value of 0.96. Cross-sectional parasite surveys The papers by Macdonald [19] , Pull and Grab [14] and a recent review of papers that reported both the EIR and the PR since 1980 by Hay et al . [54] were used as a basis to find any papers that reported both the EIR and PRs highly stratified by age. Additional papers were found by searching bibliographies of the existing publications. Papers were also identified through a PubMed search using the terms 'prevalence' or 'parasite rate' and 'entomological inoculation rate' or 'human biting rate.' Papers were included if they reported the PR stratified in at least two age classes in children <2 years. New papers were identified periodically after the search and added to the list. For each one of the 23 studies, data were extracted and the likelihood computed at the highest level of stratification reported. Simple catalytic models [14] were fitted to the data to get a crude estimate of the FOI from the PR ( X ) as a function of age: It was assumed that r =0.005 per day. In Equation 1, time and the index of heterogeneous biting always appear together, so they are not identifiable. Moreover, cross-sectional surveys do not have a fixed time interval, because exposure accumulates with age. The index of heterogeneous biting was therefore fixed at the fitted value from the Saradidi study (that is, α ≈4.6) and the parameter describing time was allowed to vary. The initial best-fit value of b was also fitted initially, but the initial fitted value was non-sensically larger than one. The parameter b was then fixed at the value from the experimental challenge studies (that is, b =0.55), and the parameter describing the time interval was fit to the scatter plot of the EIR versus transmission efficiency ( Fig. 3 ). Cross-sectional serological and parasitological surveys The original data from the study described by Corran et al . [34] were reanalysed to estimate both the SCR and the FOI. Analysis of SCR also uses Equation 5, but different parameter names are typically used for the SCR ( λ ) and the FOI ( h ), and for the decay rate of seropositivity ( ρ ) rather than parasite clearance rates ( r ). Malaria parasites are not transmitted vertically, from mother to child, but maternal antibodies are often present in infants, so our estimates of the SCR ignored infants. Longitudinal studies A search for other longitudinal studies was undertaken using the terms 'malaria incidence' and 'entomological inoculation rate' and 'longitudinal' or 'force of infection' and 'entomological inoculation rate' and 'longitudinal.' No additional papers were found in this way. Later, two other papers were discovered in other ways and added to the analysis [36] , [37] . In the Garki study, estimates of the human biting rate were reported, the number of bites by potential vectors per person per day. Estimates of the EIR were made by assuming that the sporozoite rate, the fraction of infectious mosquitoes, was 2.5%, with a range between 1 and 5%. The plotted data from Dielmo included only children <7 years. How to cite this article: Smith, D. L. et al . A quantitative analysis of transmission efficiency versus intensity for malaria. Nat. Commun. 1:108 doi: 10.1038/ncomms1107 (2010).